Suppression of the FOXM1 transcriptional programme via novel small molecule inhibition The transcription factor FOXM1 binds to sequence-specific motifs on DNA (C/TAAACA) through its DNA-binding domain (DBD) and activates proliferation- and differentiation-associated genes. Aberrant overexpression of FOXM1 is a key feature in oncogenesis and progression of many human cancers. Here—from a high-throughput screen applied to a library of 54,211 small molecules—we identify novel small molecule inhibitors of FOXM1 that block DNA binding. One of the identified compounds, FDI-6 (NCGC00099374), is characterized in depth and is shown to bind directly to FOXM1 protein, to displace FOXM1 from genomic targets in MCF-7 breast cancer cells, and induce concomitant transcriptional downregulation. Global transcript profiling of MCF-7 cells by RNA-seq shows that FDI-6 specifically downregulates FOXM1-activated genes with FOXM1 occupancy confirmed by ChIP-PCR. This small molecule-mediated effect is selective for FOXM1-controlled genes with no effect on genes regulated by homologous forkhead family factors. Evidence is accumulating to implicate deregulation of transcription factor networks as a major pathogenic event in many human cancers [1] , [2] , [3] . In healthy cells, transcription factors control the spatial and temporal conversion of DNA-encoded information into functional RNAs and proteins, thereby directing complex signalling pathways crucial to cellular function [4] , [5] . In cancer, mutations in upstream regulators, aberrant gene amplification and further perturbations resulting from such changes may destabilize proper function of the transcription factor network and drive disease [6] , [7] , [8] . There is a need for tools to intervene directly with transcription factors to dissect how the complex feedback and regulatory mechanisms work in a healthy context, and to evaluate the potential for exploiting these targets therapeutically. Small molecule intervention is a particularly attractive avenue to address both of these points [9] , [10] , [11] . First, ligands can be designed with favourable pharmacokinetic properties or modified to provide spatiotemporal delivery. Second, ligands tailored to specific domains or interfaces that minimize off-target effects may then be employed as tools to further interrogate the target’s biological function. Unfortunately, transcription factors outside the nuclear receptor family lack substrate-binding pockets, are often characterized by hydrophobic surfaces with few druggable regions and have historically proven difficult targets [12] . Past efforts to perturb transcriptional pathways have therefore focused on known protein–protein interfaces or particular recognition elements on DNA. Notable examples include distamycin-inspired polyamides, which recognize the DNA minor groove in a sequence-specific manner, and have successfully been applied to disrupt assembly of general transcription machinery at those loci [13] . Peptidomimetics, such as the stapled α-helix BCL-2 domains, have generated protease-resistant, cell-permeable tools to antagonize protein dimerization and induce selective activation of apoptotic pathways in cancer cells [14] . Such a strategy might be applied to disrupt transcription factor interactions with promoter DNA. In addition, a recent publication reports a novel small molecule that directly binds to the oncogenic transcription factor ETV1 and inhibits its transcriptional activity [15] . The transcription factor FOXM1 regulates a network of proliferation-associated genes critical to mitotic spindle assembly [16] , chromosome segregation [17] and G2/M transition [18] , with depletion leading to cell cycle arrest. Importantly, aberrant upregulation of FOXM1 has been shown to be a key driver of cancer progression and has been proposed as an initiating factor of oncogenesis [3] , [19] , [20] . Furthermore, FOXM1 overexpression has been implicated in the development of chemotherapeutic resistance in human breast cancer [21] , [22] , where high protein levels correlate with poor clinical outcome [23] , [24] and the endogenous level of FOXM1 has been suggested as a general diagnostic biomarker for cancer progression [25] . Thus, inhibition of FOXM1 activity is an attractive goal for cancer therapy. FOXM1 functions as a gene-specific transcriptional activator by binding to DNA consensus sequences through a highly conserved and well-characterized DNA-binding domain (DBD) [26] . Although such an interface has been recognized as an enticing target, the absence of small molecules known to bind FOXM1 makes structure-based rational design of drug candidates challenging [27] . Previously, others have shown that the natural product thiostrepton inhibits the transcriptional activity of FOXM1 (refs 28 , 29 ). We demonstrated that the ligand makes direct contact with FOXM1 and inhibits DNA binding in cells [30] . However, thiostrepton is a promiscuous molecule with potent off-target effects, most notably inhibition of the 20S proteasome [31] and arrest of mitochondrial protein synthesis [32] . Thus, thiostrepton cannot be used to elucidate the primary effects caused by the inhibition of FOXM1 binding to DNA [33] . We designed and exploited a robust, biophysical high-throughput screening (HTS) assay to identify inhibitors of FOXM1 that block DNA binding. We discovered an inhibitor that blocks FOXM1 binding to DNA in human cancer cells and suppresses the transcription of genes under FOXM1 control. FOXM1–DBD associates with consensus motif To interrogate binding of FOXM1 to its consensus DNA duplex, we designed a fluorescence polarization (FP) assay ( Fig. 1a ). In this system, association or dissociation of fluorophore-labelled DNA duplex to FOXM1 protein can be monitored as a function of linear and perpendicular polarization [34] . We generated a 16-bp double-stranded DNA (dsDNA) probe containing repeats of the known FOXM1 recognition motif (T/CAAACA) and a single 6-carboxyfluorescein label ligated to the 5′-end of the forward strand. Recombinant FOXM1–DBD, a truncated fusion product containing only the winged helix domain (aa 222–360), was titrated with dsDNA probe and examined by FP, which demonstrated that FOXM1 DBD associates with the DNA probe in a dose-dependent manner with K d =224±30 nM ( Fig. 1b ). This FOXM1 DBD construct has been previously identified as the minimal component of the canonical FOXM1–DNA-binding mode [26] . Notably, the dissociation constant for this truncated form of the protein for its 16 bp DNA consensus target is in good agreement with that of the full-length protein as determined by FP ( K d =300±64 nM, Supplementary Fig. 1 ) or by electrophoretic mobility shift assay (EMSA) [30] . Thus, we employed FOXM1 DBD to discover novel inhibitors of DNA binding. 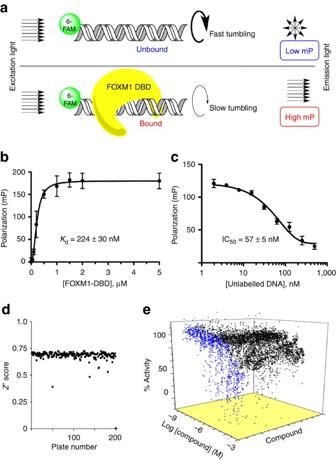Figure 1: Design of FP assay to screen for inhibitors of FOXM1–DNA binding. (a) Schematic of FP assay principle. Polarized light excites the fluorophore-labelled DNA consensus sequence probe. The proportion of polarized light recovered on emission is related to the total mass of the probe, thus binding of probe and FOXM1 DBD can be monitored. (b) FP reports binding of FOXM1 DBD with tagged consensus DNA. (c) Unlabelled consensus DNA efficiently displaced tagged DNA in a dose-dependent manner. A large signal window (>100 mP) between bound and unbound states indicated a robust assay. (d)Z’ score for each plate in screen. AggregateZ’ score was 0.71, indicating a highly robust assay. (e) Waterfall plot showing dose–response curves for 170 active and 907 inconclusive hits in blue and black, respectively. Data are reported as average of replicates (n=3) and error bars indicate s.d. throughout the figure. Figure 1: Design of FP assay to screen for inhibitors of FOXM1–DNA binding. ( a ) Schematic of FP assay principle. Polarized light excites the fluorophore-labelled DNA consensus sequence probe. The proportion of polarized light recovered on emission is related to the total mass of the probe, thus binding of probe and FOXM1 DBD can be monitored. ( b ) FP reports binding of FOXM1 DBD with tagged consensus DNA. ( c ) Unlabelled consensus DNA efficiently displaced tagged DNA in a dose-dependent manner. A large signal window (>100 mP) between bound and unbound states indicated a robust assay. ( d ) Z ’ score for each plate in screen. Aggregate Z ’ score was 0.71, indicating a highly robust assay. ( e ) Waterfall plot showing dose–response curves for 170 active and 907 inconclusive hits in blue and black, respectively. Data are reported as average of replicates ( n =3) and error bars indicate s.d. throughout the figure. Full size image Titration of a pre-bound complex of FOXM1 DBD and labelled dsDNA probe with increasing amounts of unlabelled dsDNA probe demonstrated the reversibility and specificity of the association ( Fig. 1c ). As expected, the IC 50 of this displacement (57±5 nM) was near the concentration of the labelled probe (50 nM), indicating that the 5′-carboxyfluorescein tag did not affect protein binding. Furthermore, thiostrepton, a previously identified inhibitor of FOXM1–DNA binding, disrupted the FOXM1 DBD–DNA interaction in gel shift assays with IC 50 =45.0±16.4 μM ( Supplementary Fig. 2 ), in good agreement with previously reported values using full-length FOXM1, IC 50 =42.6±1.4 μM (ref. 30 ). Screening assay for inhibitors of FOXM1-DNA To identify inhibitors of FOXM1–DNA binding, we developed a high-throughput screen based on the perturbation of FOXM1 DBD—DNA complex measured by FP (ref. 35 ). Minor adjustments were made to the assay as presented above ( Fig. 1c ), to provide suitability for a HTS protocol in 1,536-well plate format. The assay buffer was supplemented with 0.01% Tween-20 and 0.1 mg ml −1 BSA to facilitate robotic dispensing, stabilize the FOXM1 DBD protein and minimize hydrophobic aggregation of material on plastic. An apparent K d value of 158 nM was calculated for binding of FOXM1 DBD to the 16-bp DNA in 384-well plate format, showing good agreement with previous values from the initial FP runs ( Supplementary Fig. 3A ). The concentration of 400 nM FOXM1 DBD was chosen for subsequent experiments, which resulted in an average window of 135 mP units between bound and unbound signals in 1,536-well plate format ( Supplementary Fig. 3B ). Pipetting was simplified into two robotic dispense steps: 3 μl 1.3 × FOXM1 DBD+1 μl 4 × DNA probe. In calibration runs with the high-throughput format, the signal-to-background ratio was ~3.2 and the Z ’ factor was 0.77. The Z ’ factor quantifies the statistical significance of the difference between positive and negative controls. A value above 0.5 indicates that more than 12 s.d. separate the bound and unbound controls; therefore, 0.77 is well within the norm for a robust assay. Identification of small molecule inhibitors of FOXM1–DNA A collection of small molecules was screened at five concentrations ranging from 0.46 μM to a maximum of 115 μM. The screening library comprises a total of 54,211 compounds assembled at the National Center for Advancing Translational Sciences. It consists of diverse drug-like molecules that provide a starting point for medicinal chemistry lead development. Compounds with annotated pharmacology including the NCGC Pharmaceutical Collection and the Tocris Biosciences diversity library were also included for potential repurposing [36] . FOXM1 DBD was first dispensed into wells and compounds (23 nl at each concentration) were transferred with a Kalypsys 1,536-pin tool. After 15 min pre-incubation, the DNA probe was dispensed and the mixture was incubated for a further 30 min before reading FP signal. The assay reported consistently high Z ’ factors (average=0.71) throughout all plates in the screen ( Fig. 1d ). Furthermore, a suitably low active (compounds with max inhibition >60%) hit rate of 0.32% suggested a useful screen and the existence of a druggable interaction. The normalized dose response data for all positive hits from the HTS are displayed as a waterfall plot in Fig. 1e , with 170 active molecules shown in blue. All 170 active molecules from initial screening were checked for reproducibility and retested in the same assay, validating 86 of the original active molecules. Active molecules that exhibited poor reproducibility, bad dose–response profile, nonspecific DNA-binding activity (hits in thiazole orange displacement counter screen), or were found to disrupt the FP assay (fluorescent artefacts or quenchers) were eliminated [37] . Ultimately, 16 Forkhead Domain Inhibitory compounds (renamed FDI-(1–16), structures provided in Supplementary Fig. 4 ) were selected for further analysis. Orthogonal EMSAs validate six active FDI compounds EMSA was chosen as an orthogonal assay to further evaluate FDI-(1–16) in dose–response. The binding of FOXM1 DBD is detected by EMSA ( K d =301±21 nM, Fig. 2a ) and is near the value reported by FP ( K d =224±30 nM, Fig. 1b ). To examine the effect of the inhibitors, FOXM1 DBD was incubated with increasing concentrations of ligand for 1.5 h at room temperature (RT), target DNA was added, electrophoresis was performed and DNA probe bands were visualized by fluorescence imaging. In this assay, 6 of the 16 FDI compounds exhibited dose-dependent inhibition of the FOXM1 DBD–DNA-binding interaction ( Fig. 2b , representative gels provided in Supplementary Fig. 6 ), confirming their activity in the primary FP screen. The remaining compounds were inactive below 200 μM; these were presumed to be false positives in the FP assay and discarded. Values were also determined for 50% growth inhibition after 72 h ligand treatment (GI 50 ) in MCF-7 breast cancer cells, which highly express FOXM1 ( Fig. 2b , inset and Supplementary Fig. 6 ). FDI-6 (3-amino- N -(4-fluorophenyl)-6-(thiophen-2-yl)-4-(trifluoromethyl)thieno[2,3-b]pyridine-2-carboxamide TFA) was the most potent EMSA-validated compound, with a representative EMSA image shown in Fig. 2c . In addition, the concordance between GI 50 and IC 50 values for FDI-6 is indicative of minimal off target activity. Furthermore, two compounds ( FDI-6 and FDI-10 ) exhibited potent IC 50 values (22.5±12.3 and 34.36±11.2 μM, respectively) comparable to that of thiostrepton (IC 50 =45.0±16.4 μM, see Supplementary Fig. 2 ). It was noteworthy that the top three validated compounds by potency— FDI-6 , FDI-10 and FDI-11 —shared a common core structure ( Fig. 2d ) suggestive of a potential pharmacophore. 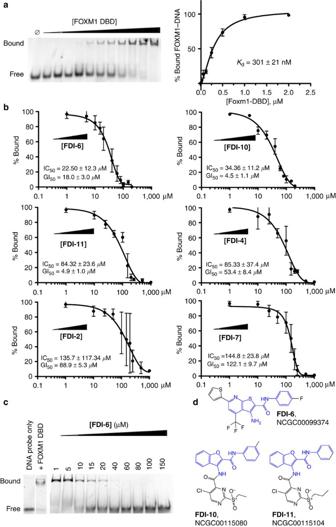Figure 2: EMSA assay provides orthogonal biophysical validation of 16 lead compounds from FP screen. (a) Representative EMSA image shows the association of FOXM1 DBD with its fluorescently tagged DNA consensus. Binding curve for the FOXM1 DBD–DNA interaction was determined by quantification of EMSA replicates. (b) Quantification of EMSA bands confirmed 6 of the 20 lead compounds selected from the FP results inhibited FOXM1–DNA binding. In rank order of potencies:FDI-6>FDI-10>FDI-11>FDI-4>FDI-2>FDI-7. Representative gel images are provided inSupplementary Fig. 5. Each inset lists the IC50as well as 72 h GI50concentrations in MCF-7 cells. (c) Representative EMSA showing the inhibitory effect ofFDI-6on the FOXM1 DBD–DNA complex. (d) Structures ofFDI-6,FDI-10andFDI-11, the most potent of the validated hit compounds, which all contain a common core structural element (highlighted in blue). Data are reported as average of replicates (n=3) and error bars indicate s.d. throughout figure. Figure 2: EMSA assay provides orthogonal biophysical validation of 16 lead compounds from FP screen. ( a ) Representative EMSA image shows the association of FOXM1 DBD with its fluorescently tagged DNA consensus. Binding curve for the FOXM1 DBD–DNA interaction was determined by quantification of EMSA replicates. ( b ) Quantification of EMSA bands confirmed 6 of the 20 lead compounds selected from the FP results inhibited FOXM1–DNA binding. In rank order of potencies: FDI-6 > FDI-10 > FDI-11 > FDI-4 > FDI-2 > FDI-7 . Representative gel images are provided in Supplementary Fig. 5 . Each inset lists the IC 50 as well as 72 h GI 50 concentrations in MCF-7 cells. ( c ) Representative EMSA showing the inhibitory effect of FDI-6 on the FOXM1 DBD–DNA complex. ( d ) Structures of FDI-6 , FDI-10 and FDI-11 , the most potent of the validated hit compounds, which all contain a common core structural element (highlighted in blue). Data are reported as average of replicates ( n =3) and error bars indicate s.d. throughout figure. Full size image FDI-6 binds FOXM1 and displaces protein from target genes Nonspecific DNA recognition by the small molecule hits was already ruled out by the thiazole orange counterscreen (see earlier). It was then important to confirm that our shortlisted hits ( FDI-6 , FDI-10 and FDI-11 ) act via direct interaction with the protein, which we achieved by native mass spectrometry. FOXM1 protein is accurately detected by this method and exists as a dimer in solution, as is frequently observed for glutathione S -transferase (GST) fusions [38] . Hit compounds FDI-6 , FDI-10 and FDI-11 were each found to bind directly to FOXM1 protein with a 1:1 stoichiometry ( Fig. 3a ). We also tested FDI-9, a compound that was active in the primary FP assay, but failed to inhibit FOXM1–DNA by EMSA, and showed that, in contrast, it does not interact with the protein. This finding supports the use of EMSA as an orthogonal assay to flag artefacts and indirect inhibitors. 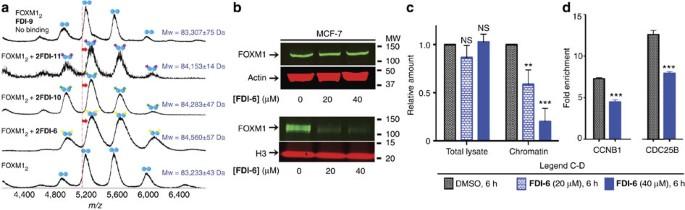Figure 3: Compound FDI-6 shows promising FOXM1-specific inhibitory effects in MCF-7 cells. (a) FDI compounds were investigated for direct interaction with FOXM1 protein by non-denaturing nano-electrospray ionization massspectrometry. EMSA-validated hitsFDI-6(yellow stars),FDI-10(green stars) andFDI-11(purple stars) associate with the protein in a 1:1 stoichiometric ratio. Negative control FDI-9 was identified as a false positive by EMSA assay and does not associate with the protein. Mass shifts indicating ligand association are indicated by red arrows. (b) Western blottings on the whole cell and chromatin fractions revealed a specific displacement of DNA bound FOXM1, while total levels were unaffected. Total MCF-7 cell lysate and chromatin bound fractions were isolated after 6 h treatment withFDI-6or DMSO control. (c) Quantification of western blottings revealed displacement of FOXM1 from DNA. Data were normalized to Actin (total lysate) and Histone H3 (chromatin fraction). (d) Targeted ChIP-PCR revealed 6 h treatment withFDI-6decreased FOXM1 occupancy at known FOXM1 target genes. Refer to legend forc,d. Data are reported as average of replicates (n=3) and error bars indicate s.d. throughout the figure. In each case, the statistical significance was determined by Student’st-test (*P<0.05, **P<0.01, ***P<0.001). Figure 3: Compound FDI-6 shows promising FOXM1-specific inhibitory effects in MCF-7 cells. ( a ) FDI compounds were investigated for direct interaction with FOXM1 protein by non-denaturing nano-electrospray ionization massspectrometry. EMSA-validated hits FDI-6 (yellow stars), FDI-10 (green stars) and FDI-11 (purple stars) associate with the protein in a 1:1 stoichiometric ratio. Negative control FDI-9 was identified as a false positive by EMSA assay and does not associate with the protein. Mass shifts indicating ligand association are indicated by red arrows. ( b ) Western blottings on the whole cell and chromatin fractions revealed a specific displacement of DNA bound FOXM1, while total levels were unaffected. Total MCF-7 cell lysate and chromatin bound fractions were isolated after 6 h treatment with FDI-6 or DMSO control. ( c ) Quantification of western blottings revealed displacement of FOXM1 from DNA. Data were normalized to Actin (total lysate) and Histone H3 (chromatin fraction). ( d ) Targeted ChIP-PCR revealed 6 h treatment with FDI-6 decreased FOXM1 occupancy at known FOXM1 target genes. Refer to legend for c , d . Data are reported as average of replicates ( n =3) and error bars indicate s.d. throughout the figure. In each case, the statistical significance was determined by Student’s t -test (* P <0.05, ** P <0.01, *** P <0.001). Full size image To determine whether an inhibitor of FOXM1–DNA in vitro could inhibit transcription factor binding in MCF-7 breast cancer cells, which highly express FOXM1 (ref. 39 ), we selected the most potent ligand FDI-6 for follow-up experiments. On isolating the nuclear fractions of FDI-6 -treated MCF-7 cells by centrifugation, western blottings revealed that a 6 h dose of 20 μM FDI-6 —approximately the biophysical IC 50 of the ligand for disrupting the FOXM1–DNA interaction—decreased chromatin-bound FOXM1 by nearly 50%, while the overall amount of FOXM1 protein was unaffected ( Fig. 3b,c ). Importantly, and in contrast to reports for thiostrepton [40] , FDI-6 did not inhibit the 20S proteasome as determined by a standard proteasome assay ( Supplementary Fig. 7 ). The observation that FDI-6 displaces FOXM1 from chromatin led us to initially investigate its effect on the gene targets CCNB1 and CDC25B (refs 6 , 16 ). Activation of these target genes has been attributed to the oncogenic potential of FOXM1, and depletion of FOXM1 reduced colony formation of acute myeloid leukemia cells due to inhibition of CCNB1 and CDC25B expression [41] . Importantly, direct occupancy of FOXM1 at its consensus sequence within both CCNB1 and CDC25B promoter regions activates transcription in reporter assays [42] . Thus, these were ideal targets to initially test the ability of FDI-6 to disrupt FOXM1–DNA in the cell. To first examine FOXM1 occupancy in these regions, we performed chromatin immunoprecipitation (ChIP) with FOXM1 antibody followed by quantitative real-time PCR (qRT–PCR) amplification of the bound DNA. This revealed a −0.68 and −0.64 log2 fold decrease in FOXM1 occupancy at CCNB1 and CDC25B gene promoters, respectively ( Fig. 3d ). The changes at specific genomic loci will not necessarily match the average global change quantitatively, as there is a context dependence for transcription factor binding [43] , [44] . However, the magnitudes of changes observed here generally agree with those reported by the chromatin blotting experiments ( Fig. 3b,c ). RNA-seq signature of FDI-6 associated with FOXM1 repression As FOXM1 is a pure transcriptional activator [45] , [46] , [47] , we expect that its displacement from gene targets should lead to specific downregulation of those gene transcripts. The ability of FDI-6 to displace FOXM1 from two established genomic targets led us to investigate the global transcriptional effects of ligand treatment rigorously by genome-wide RNA sequencing (RNA-seq). We thus examined the effect of FDI-6 treatment on RNA transcript levels in MCF-7 cells at 3, 6 and 9 h time points. The experiment was performed in triplicate at each of the three time points and the untreated control. 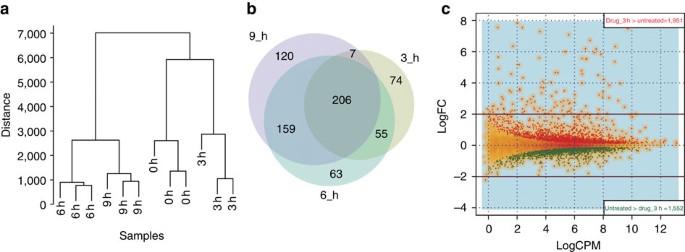Figure 4: Genome-wide RNA-seq shows that FDI-6 treatment selectively downregulates transcription of FOXM1 target genes. (a) Hierarchical clustering of gene expression profiles, showing the similarity of different treatment times. SeeSupplementary Table S2for details of Euclidian distance between paired libraries. (b) Venn diagrams showing the overlap of differentially expressed genes at the different time points. (c) Global differential expression map of RNA-seq after 3 h treatment versus untreated.yaxis: logarithm of fold change (logFC);xaxis: logarithm of counts per million of reads (logCPM). Red dots: upregulated genes (n=1,951); green dots: downregulated genes (n=1,552). Figure 4a shows the hierarchical clustering of gene expression profiles demonstrating that independent replicates at each time point group together and that their expression profiles show strong reproducibility. Furthermore, a substantial core set of 206 genes are found to be differentially expressed at each treatment time point, indicating agreement between samples ( Fig. 4b , GEO: GSE58626 and differential expression is provided as Supplementary File ). Figure 4c shows a single replicate of differentially expressed genes after 3 h with up (red) and down (green) genes plotted by the logarithm of fold change (logFC, y axis) and logarithm of counts per million reads ( x axis). Figure 4: Genome-wide RNA-seq shows that FDI-6 treatment selectively downregulates transcription of FOXM1 target genes. ( a ) Hierarchical clustering of gene expression profiles, showing the similarity of different treatment times. See Supplementary Table S2 for details of Euclidian distance between paired libraries. ( b ) Venn diagrams showing the overlap of differentially expressed genes at the different time points. ( c ) Global differential expression map of RNA-seq after 3 h treatment versus untreated. y axis: logarithm of fold change (logFC); x axis: logarithm of counts per million of reads (logCPM). Red dots: upregulated genes ( n =1,951); green dots: downregulated genes ( n =1,552). Full size image We expected (i) specific downregulation of FOXM1 gene targets, (ii) the activation of secondary and tertiary downstream responses to changes in the primary gene targets and (iii) non-FOXM1-specific, differentially expressed genes responding to the stress of ligand treatment. Table 1 presents the most significant ( P <10 −14 ) Gene Ontology terms for differentially expressed genes after ligand treatment. Importantly, cell cycle regulation and mitotic processes, of which FOXM1 is a known activator, are significantly downregulated. After 6 h, CCNB1 is decreased −0.86 (log2 fold change, P =1.9 × 10 −42 ) and CDC25B is decreased −0.36 ( P =4.3 × 10 −12 ). These values closely correlate with the fraction of FOXM1 that is displaced in ChIP–PCR ( Fig. 3c ) and also agree with downregulation reported by separate qPCR validation runs after the same treatment ( Supplementary Fig. 8 ). Many other established transcriptional targets of FOXM1 (ref. 27 ) were also strongly downregulated by FDI-6 at each of the treatment time points. Measured at 6 h, these include CCNA2 (−0.65, P =2.6 × 10 −27 ), CDKN3 (−0.739, P =3.1 × 10 −13 ), CENPA (−0.61, P =8.3 × 10 −15 ), KIF20A (−1.22, P =1.1 × 10 −95 ), NEK2 (−0.86, P =3.3 × 10 −16 ), PLK1 (−0.92, P =3.2 × 10 −63 ) and AURKA (−0.83, P =1.4 × 10 −50 ) and compared in magnitude with changes seen following small interfering RNA (siRNA) knockdown reported by Wonsey et al. [16] Table 1 Gene Ontology signature of FDI-6. Full size table A FOXM1 inhibitor should exhibit this phenotype in any cell line expressing FOXM1. To rule out a cell-specific explanation for the response of estrogen receptor-positive MCF-7 cells to FDI-6 , we examined two additional patient-derived malignant adenocarcinoma cell lines commonly used in the literature: MDA-MB-231 ER-negative breast and PEO-1 ovarian cancer cells, which both highly express FOXM1 (refs 39 , 48 ). Both of these additional cell lines were sensitive to FDI-6 in cell viability assays (GI 50 =21.8 and 18.1 μM, respectively) and exhibited comparable downregulation of CDC25B after a 3-h treatment with the molecule ( Fig. 5 ). This finding supports the proposed mechanism of action of FDI-6 as an inhibitor of FOXM1 binding and suggests its utility across multiple cellular systems expressing the transcription factor. 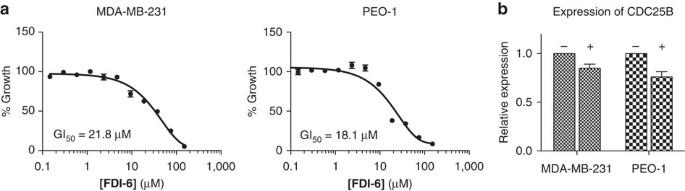Figure 5: FDI-6 retains activity in MDA-MB-231 and PEO-1 adenocarcinoma cell lines. (a) Seventy-two hours treatment withFDI-6shows dose-dependent effect on cell growth in MDA-MB-231 and PEO-1 breast and ovarian cancer cell lines. (b) FDI-6 downregulates CDC25B expression after 3 h treatment. Figure 5: FDI-6 retains activity in MDA-MB-231 and PEO-1 adenocarcinoma cell lines. ( a ) Seventy-two hours treatment with FDI-6 shows dose-dependent effect on cell growth in MDA-MB-231 and PEO-1 breast and ovarian cancer cell lines. ( b ) FDI-6 downregulates CDC25B expression after 3 h treatment. Full size image FDI-6 effect is specific for genes with FOXM1 occupancy A critical property of a bona fide FDI ligand, according to our model, would be the downregulation of genes immediately downstream of FOXM1-occupied promoters. In contrast, genes that lack FOXM1 occupancy in the promoter should not be differentially expressed as a result of such a ligand, but may respond to downstream effects caused by changes in FOXM1-responsive genes. The identification of several established FOXM1 targets here supports FDI-6 as a FOXM1 inhibitor. To further characterize the entire population of differentially expressed genes, we examined their correlation with FOXM1 promoter occupancy. Using the publicly available ENCODE FOXM1 ChIP-seq data set in MCF-7 cells, we determined the abundance of verified FOXM1 protein-binding sites within the up- and downregulated sets of differentially expressed genes ( Fig. 6a , top panel). This analysis revealed a highly significant ( P <1 × 10 −16 ) 19-fold enrichment of FOXM1-binding sites exclusively in the downregulated set. In contrast, the upregulated differentially expressed genes were not significantly enriched ( P >0.005) for promoter FOXM1-binding sites over the background of genes not differentially expressed. Motif analysis of FOXM1-binding peaks reported the consensus sequence used to identify FDI-6 originally (T/CAAACA, E -value=2.5 × 10 −62 , Supplementary Fig. 9 ), and ligand treatment specifically downregulated these FOXM1-activated genes, providing strong evidence that the inhibitory effect of FDI-6 on FOXM1 binding translates into cells. 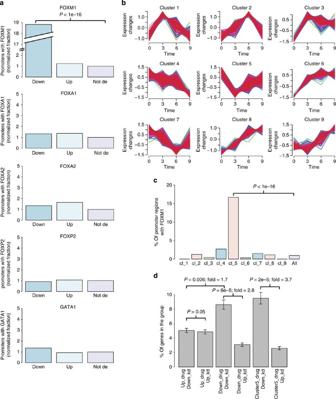Figure 6: Differential expression signature of FDI-6 is associated with FOXM1 promoter occupancy and siRNA FOXM1. (a) Bar plots showing the percentage of differentially expressed gene sets with a transcription factor occupancy in the promoter region (2 kb upstream of transcription start site (tss)). Plots are shown for the closely related forkhead transcription factors FOXM1, FOXA1, FOXA2 and FOXP2, as well as the transcriptional activator GATA1. For each plot, from left to right, bars represent downregulated (down), upregulated (up) and not differentially expressed (not de) gene sets. (b) Temporal cluster analysis grouping genes that show similar changes in expression afterFDI-6treatment. (c) Bar plot showing the percentage of genes in the different temporal clusters with a FOXM1 peak in the promoter region. (d) Bar plot showing the fraction of genes that were up- and downregulated byFDI-6and were commonly differentially expressed in an existing microarray data set of FOXM1 siRNA knockdown. Error bars indicate s.e.m. Figure 6: Differential expression signature of FDI-6 is associated with FOXM1 promoter occupancy and siRNA FOXM1. ( a ) Bar plots showing the percentage of differentially expressed gene sets with a transcription factor occupancy in the promoter region (2 kb upstream of transcription start site (tss)). Plots are shown for the closely related forkhead transcription factors FOXM1, FOXA1, FOXA2 and FOXP2, as well as the transcriptional activator GATA1. For each plot, from left to right, bars represent downregulated (down), upregulated (up) and not differentially expressed (not de) gene sets. ( b ) Temporal cluster analysis grouping genes that show similar changes in expression after FDI-6 treatment. ( c ) Bar plot showing the percentage of genes in the different temporal clusters with a FOXM1 peak in the promoter region. ( d ) Bar plot showing the fraction of genes that were up- and downregulated by FDI-6 and were commonly differentially expressed in an existing microarray data set of FOXM1 siRNA knockdown. Error bars indicate s.e.m. Full size image We further applied this methodology to examine the specificity of FDI-6 for FOXM1 over other Forkhead Box (FOX) proteins, which have highly homologous DBDs. We reanalysed the RNA-seq signature of FDI-6 for enrichments in ChIP-seq-binding peaks of all related forkhead factors for which available ENCODE data sets exist: FOXA1, FOXA2 and FOXP2 ( Fig. 6a , middle three panels). Remarkably, despite the >60% conservation among residues comprising the DBDs of FOX family transcription factors and the similarity of their consensus sequence motifs [49] , genes differentially expressed after FDI-6 treatment did not show enrichment over background for promoter occupancy of any other FOX transcription factors. This finding supports the specificity of the ligand for FOXM1 DBD over similar forkhead DBDs. Likewise, we show that there is no enrichment for sites of GATA1 occupancy ( Fig. 6a , bottom panel). This latter comparison shows that the effect of the molecule is not associated with a general suppression of transcriptional activity, but is specific for the FOXM1 transcriptional programme. To further characterize the effects of FDI-6 on the FOXM1 transcriptional programme, we sorted sets of differentially expressed genes into groups based on their response profiles during the three treatment times. Our reasoning was that genes directly affected by FOXM1 occupancy would respond relatively quickly and consistently to displacement of FOXM1. This methodology, called time-point cluster analysis, identified a set of 208 genes that are immediately downregulated after FDI-6 treatment (Cluster 5, Fig. 6b , cluster assignment of each gene is provided in Supplementary File ). Inhibition of FOXM1–DNA should immediately downregulate FOXM1-activated genes; thus, we expect that Cluster 5 should correlate best with promoter FOXM1 occupancy. Indeed, Cluster 5 is enriched 17-fold ( P =5 × 10 −82 ) over the background for genes with promoter FOXM1-binding sites ( Fig. 6c ). Importantly, no other clusters exhibited significant enrichment ( P <0.005) of genes with FOXM1-binding sites. Furthermore, each of the FOXM1 target genes discussed above is present within this cluster. This finding supports the notion that FDI-6 induces a specific response of FOXM1 inhibition and that additional transcriptional responses represent downstream secondary effects of downregulated primary FOXM1 targets or of nonspecific ligand stress. We remarked above that a number of the representative genes downregulated by FDI-6 were similarly decreased following siRNA knockdown of FOXM1 (ref. 16 ). We can explore this association across the entire transcriptome, as a highly specific compound should induce a similar differentially expressed gene signature to siRNA knockdown. Using an existing microarray profile of FOXM1 knockdown in BT-20 breast cancer cells (GEO accession: GSE2222) for comparison, we observe a significant ( P =6 × 10 −5 ) overlap with the FDI-6 gene signature ( Fig. 6d ). This reveals a tendency for genes downregulated by siRNA FOXM1 to be similarly downregulated by the compound. In contrast, there is no significant ( P >0.05) correlation between the genes upregulated by the two treatments. Furthermore, the trend is even more pronounced within the subset of genes in Cluster 5, which are 3.7-fold ( P =2 × 10 −5 ) enriched for genes downregulated by siRNA FOXM1. Lastly, it is a notable distinction that the small molecule acts directly on the DNA-binding activity of FOXM1 and the phenotype arises after only 3 h treatment, in contrast to the 48-h incubation time needed to degrade FOXM1 protein by RNA interference. Taken together, these series of analyses show that FDI-6 specifically inhibits FOXM1 association with consensus sequence DNA targets and prevents downstream transcriptional activation of these targets in cells, without inhibiting the related forkhead factors or perturbing FOXM1 protein level. We have identified small molecule inhibitors that disrupt FOXM1–DNA interaction using an assay based on the FP response of a labelled consensus oligonucleotide bound to recombinant FOXM1 DBD protein. From a library of 54,211 structurally diverse ligands, we identified 6 FDI compounds that were cross-validated in orthogonal binding assays. Notably, three of these compounds exhibit a common pharmacophore, suggesting a common structural mechanism. We further characterized the lead inhibitor NCGC00099374 ( FDI-6 ) to show that it acts by targeting FOXM1 protein and broadly represses transcription of FOXM1-activated genes by displacing FOXM1 from chromatin. This activity is reflected throughout the transcriptome and is recapitulated by a Gene Ontology summary, which indicates that entire pathways known to be controlled by FOXM1 transactivation—mitosis, nuclear division and cell cycle processes—are significantly inhibited by FDI-6 . Taken together, our data support a direct mechanism of action whereby FDI-6 blocks the binding of FOXM1 to target DNA, preventing the normal activation of FOXM1 target genes. We cannot absolutely rule out the possibility of a contribution from some unknown off-target effect(s) of FDI-6 . However, it is a significant indication of the small molecule’s specificity that despite the conserved DBD and a 71% overlap of ChIP-seq peaks for FOXM1 and FOXA1 (ref. 44 ), genes repressed by FDI-6 are exclusively targets of FOXM1 and not of FOXA1 or related forkhead factors. An inhibitor with the ability to globally disrupt association of FOXM1 with DNA consensus sites in cells provides a valuable tool to probe FOXM1 occupancy. Previously, the ability to interrogate or intervene with the direct consequences of transcription factor binding has been limited. We previously reported that thiostrepton, a natural product antibiotic, binds directly to FOXM1 in cells and downregulates target gene expression [30] . However, the use of thiostrepton is confounded by its inhibition of the 20S proteasome. Thiostrepton also induces significant toxicity (GI 50 =2.7 μM) well below the concentration needed to affect FOXM1 inhibition (IC 50 =45.0±16.4 μM). These peripheral activities of thiostrepton introduce some uncertainty about its dominant mechanism of action in cells and thus cannot be used to unambiguously probe FOXM1. In contrast, the novel inhibitor FDI-6 is inactive against the proteasome, and concordance between its biophysical IC 50 and cellular GI 50 values (22.5±12.3 and 18.0±3.0 μM, respectively) suggests it does not suffer from the off-target effects of thiostrepton. The characteristics of smaller molecular size, greater aqueous solubility and a scaffold amenable to future optimization are further advantages to the novel molecule. We have also provided evidence for FDI-6 -mediated downregulation of established FOXM1-controlled genes. By way of comparison, the same gene targets— CDKN3 (−0.739, after 6 h FDI-6 ), CENPA (−0.61), KIF20A (−1.22) and NEK2 (−0.86), which all have strong FOXM1-binding sites in their promoters—were downregulated by the same magnitude in a previous study employing qPCR after siRNA knockdown of FOXM1 (ref. 16 ). It is significant for its utility as a specific probe of FOXM1 occupancy that FDI-6 stimulates a comparable transcriptional response after only 3 h and without ablating FOXM1 protein. The genome-wide repression of the FOXM1 transcriptional programme by FDI-6 demonstrates a mechanistic proof-of-concept. At present, the application of FDI compounds to antagonize FOXM1–DNA provides a powerful means to probe the complex consequences of FOXM1 occupancy on transcription. Given that aberrant overexpression of FOXM1 protein is increasingly recognized as an initiating event in oncogenesis [19] , cancer progression [50] and therapeutic resistance [21] , [22] , the capacity to inhibit FOXM1–DNA with small molecules has considerable potential, which we will be exploring as part of future work. FOXM1–DBD protein preparation FOXM1–DBD complementary DNA was cloned from the human full-length FOXM1c cDNA fragment (Origene Technologies). After PCR amplification with primers containing Sgf 1 and Mlu I restriction sites, the products were gel purified and ligated in frame to the amino terminus of GST into the linear pEX-N-GST vector (Origene Technologies) containing a T7 promoter, allowing for isopropyl-β- D -thiogalactoside-inducible expression of the fusion protein. Ligated plasmids were inserted into BL21/DE3 Escherichia coli cells by heat-induced transformation. Positive clones were selected by colony PCR screening and DNA sequencing confirmed successful insertion. Cells were grown at 37 °C in Luria Broth media until reaching an optical density of 0.8 at which point the temperature was decreased to 18 °C, and GST-FOXM1 DBD expression was induced by addition of 1 mM isopropyl-β- D -thiogalactoside overnight. Culture conditions produced suitable amounts of protein (in excess of 2 mg l −1 culture medium) that purified easily with no contaminant or degradation product bands. Representative gel images of purified products are provided in Supplementary Fig. 10 . Fluorescence polarization assay Setup runs of the FP assay were performed in 96-well plates and read on a PHERAStar (BMG Labtech) with a 488/520 FP filter. The screening assay was scaled down successively to 384- and 1,536-well plate formats and read on a ViewLux high-throughput charge-coupled device imager (Perkin-Elmer, Wellesley, MA). EMSA binding tests Association of FOXM1 with 15 nM dsDNA consensus sequence oligo (forward strand: 5′-FAM-AAACAAACAAACAATC-3′) was recorded by EMSA. Protein and dsDNA components were mixed in a 20-μl reaction volume, incubated at RT for 30 min and run directly on a 6% DNA retardation gel (Sigma) for 10 min at 40 V and 20 min at 120 V. The binding buffer consists of 20 mM Tris (pH 7.5), 100 mM KCl, 1 mM EDTA, 0.1 mM dithiothreitol, 10% vol/vol glycerol, 0.010 mg ml −1 BSA. For displacement experiments, 2 μl of 10 × probe DNA was added to 18 μl of FOXM1 DBD incubated with FDI compounds for 1.5 h ([FOXM1 DBD] f =750 nM, [DNA probe] f =15 nM). After 15 min incubation time, samples were loaded directly and electrophoresis performed as above. Cell culture MCF-7, MDA-MB-231 and PEO-1 cells were obtained from the European Collection of Animal Cell Cultures. MCF-7 and MDA-MB-231 cells were grown in DMEM medium (Sigma) supplemented with 10% fetal bovine serum (Sigma). PEO-1 cells were cultured in RPMI (Invitrogen) media, also supplemented with 10% fetal bovine serum. Antibodies Rabbit polyclonal IgG FOXM1 antibody (C-20) was acquired from Santa Cruz Biotech (SC-502, lot# G2312). Actin was acquired from Abcam (AC-15, lot GR91208-03, used 1:5,000). Histone H3 antibody was acquired from Cell Signalling (4499S, lot 1, used 1:2,000). LiCor secondary antibodies were used for infrared detection using goat-anti-mouse (680LT, lot C1109-02, used 1:20,000) and goat-anti-rabbit (800CW, lot C30626-03, used 1:15,000). Full gel images for each western blotting are provided in Supplementary Fig. 11 . qRT–PCR primers Quantitect primers (Qiagen) were used for qRT–PCR including ACTB (QT00095431), CCNB1 (QT00006615), CDC25B (QT00028350) and YWHAZ (QT00087962). Native mass spectrometry Mass spectra were recorded on a Synapt HDMS instrument (Waters UK Ltd, Manchester, UK). The concentration of FOXM1 was 4 μmol dm −3 , while the final concentration of compounds after adding to the protein was 50 μmol dm −3 . All measurements were carried out in a positive ion mode. Spraying conditions were as follows: capillary voltage 1.7–1.8 kV, cone voltage 40–80 V, source temperature 20 °C, trap collision energy 12.0 V and transfer collision energy 12.0 V with trap and transfer pressure 5.31 × 10 −2 mbar, Ion Mobility spectrometry pressure 5.02 × 10 −1 mbar and Time-of-Flight analyser pressure 1.2 × 10 −6 mbar. External calibration of the spectra was achieved using caesium iodide at 100 mg ml −1 in water. Data acquisition and processing were performed using Micromass MassLynx 4.1. 20S proteasome inhibition A 20S Proteasome Activity kit (Millipore) was used to determine compound effect on proteasome activity, according to the manufacturer’s protocol. Briefly, an AMC peptide that is conditionally fluorescent on proteasome cleavage was used to generate a standard curve to determine an appropriate concentration window for the assay. A 1:200 AMC concentration was determined to give suitable signal:noise response and used in the assay. Inhibitor (10 μM) or dimethyl sulphoxide (DMSO) control, recombinant proteasome and AMC substrate were mixed and incubated at 37 °C for 90 min. Fluorescence was then read on a Pherastar (BMG) using a 380/460 filter set. Inhibitory responses were determined normalized to DMSO control and compared with a known proteasome inhibitor MG-132. Western blottings Western blotting was carried out with total lysate and chromatin-isolated fractions from MCF-7 cells treated for 6 h with FDI-6 (40 μM) or DMSO control. For total lysate preparations, cells were grown and were harvested by scraping in PBS and pelleted by centrifugation. Cell pellets were lysed with 1 ml ice-cold 1 × RIPA buffer, with protease inhibitors (Roche). The lysate was agitated for 1 h at 4 °C by end-to-end rotation; the supernatant was collected following centrifugation and lysate concentration was measured using Pierce BCA Protein Assay kit following the manufacturer’s protocol. Chromatin isolation protocol was adapted from Mendez et al. [51] To isolate chromatin, cells were resuspended in Chromation Isolation Buffer A and the cells were incubated for 5 min on ice. Nuclei were collected by low-speed centrifugation (4 m, 1,300 g at 4 °C). Nuclei were washed once in Chromatin Isolation Buffer A and then lysed in Chromatin Isolation Buffer B. Insoluble chromatin was collected by centrifugation (4 m, 1,700 g at 4 °C), washed once in Chromatin Isolation Buffer B and centrifuged again under the same conditions. The final chromatin pellet (P3) was resuspended in Laemmli buffer and sonicated for 15 s in a Tekmar CV26 sonicator using a microtip at 25% amplitude. After harvesting, 20 μl of the recovered cell samples (total lysate or chromatin isolated fraction) were loaded onto 8–16% Tris-Glycine mini gels followed by electrophoresis at 150 V for 90 min. Rapid protein transfer was accomplished using the manufacturer’s recommended 7-min protocol on the iBlot system (Invitrogen). The membrane was first washed in Odyssey block buffer (Li-Cor) three times (10 ml per wash). Primary actin antibody (total lysate control) or histone H3 antibody (chromatin isolation control) from Abcam were used at 1:5,000 and 1:10,000, respectively. The FOXM1 antibody was used at 1:1,000 dilution. Primary antibodies were incubated overnight at 4 °C. Secondary antibodies were incubated at RT for 45 min. Goat anti-mouse IRDye-680 secondary antibody was used for actin and goat anti-rabbit IR Dye-800 for FOXM1. Blottings were visualized on the Li-C or scanner, and quantification of FOXM1 relative to β-actin (total lysate) or Histone H3 (chromatin isolation) was carried out for each lane. Chromatin immunoprecipitation MCF-7 cells were grown in 15 cm 2 dishes to 70% confluence before compound or DMSO control treatment for 6 h. Cells were washed with PBS, cross-linked with 1% formaldehyde at RT for 10 min and quenched with 1/20 volume glycine (2.5 M). Cells were harvested by scraping into cold PBS containing protease inhibitors and cell pellets stored at −80 °C. Cell pellets were lysed and resuspended in buffer containing protease inhibitors. Samples were sonicated on ice using a bioruptor UCD200 sonicator (Diagenode) for 15 min at high power with a pulse of 30 s on/30 s off. Samples then supplemented with Triton X-100 to a final concentration of 1% and centrifuged at 20,000 g for 10 min at 4 °C. Protein-A dynabeads (Invitrogen) were washed with block solution (PBS plus 0.5% BSA) and incubated overnight with 3 μg FOXM1 (Sc-502) antibody in block solution, followed by washing three times in block solution. Supernatants from cell lysates were incubated overnight with antibody capture beads and then the beads were collected and washed six times with RIPA buffer II. Bound DNA was eluted by incubation at 65 °C for 16 h in ChIP elution buffer and purified using a Qiaquick PCR clean-up kit. PCR was carried out using 2 μl of purified DNA in a 20-μl reaction with Power Sybr PCR mix (ABI), using the cycle conditions: 95 °C for 10 min followed by 40 cycles of 15 s at 95 °C, 30 s at 60 °C followed by generation of a dissociation curve. Primer sequences used are as follows: 5′-AAGAGCCCATCAGTTCCGCTTG-3′ (CDC25B promoter fwd), 5′-CCCATTTTACAGACCTGGACGC-3′ (CDC25B promoter rev); 5′-CGCGATCGCCCTGGAAACGCA-3′ (CCNB1 promoter fwd), 5′-CCCAGCAGAAACCAACAGCCGT-3′ (CCNB1 promoter rev); and 5′-TGCCACACACCAGTGACTTT-3′ (CCND1 intergenic control fwd), 5′-ACAGCCAGAAGCTCCAAAAA-3′ (CCND1 intergenic control rev). Enrichment values were calculated in Excel by normalizing against cyclin D1 intergenic control. RNA-seq and analysis Samples were processed following the standard TruSeq (Illumina) protocol. Fastq files containing 100 single-end reads were processed with trim-galore ( http://www.bioinformatics.babraham.ac.uk/projects/trim_galore/ ) to perform adapter trimming and low-quality reads filtering. The filtered reads were then aligned to the human genome (hg19) with tophat2 (ref. 52 ) and transcripts were assigned to gene and counted using htseq-count ( http://www-huber.embl.de/users/anders/HTSeq/doc/overview.html ). See Supplementary Tables 1 and 2 for summary statistics. Differential expression analysis Differential expression analysis was performed using edgeR (ref. 53 ). The three replicates belonging to the different time points (3, 6 and 9 h) were tested for differential expression versus the control condition (0 h treatment), by using the exact test for differences between two groups of negative binomial counts (function exactTest in the R package ‘edgeR’). This method computes the genewise difference of counts taking into account variability across replicates. By default, the method normalizes for the total library size by calculating counts per million of reads. Genes with a false discovery rate (FDR) below 0.01 were considered significant for differential expression ( Fig. 4c ). For the overlap among differentially expressed genes shown in the Venn diagram ( Fig. 4b ), we considered only genes with FDR<0.01 and absolute logarithm of fold change (logFC)>1, that is, genes upregulated at least twofold or downregulated at least 50%. Temporal clustering The clustering of temporal profiles of gene expression was done using the R package ‘MFuzz’ [54] , which performs soft clustering of genes based on their expression values using the fuzzy c-means algorithm. We first selected only the 1,552 genes having a substantial change in either one of the time points (that is, abs(logFC) > 0.75); we then ran the fuzzy c-means algorithm with parameters 9 and 1.35, respectively, the number of clusters and the fuzzification parameter. The temporal profiles used for clustering and shown in Fig. 6b are standardized such that the average expression value for each gene in the different time points is 0 and the s.d. is 1. In the supporting.xls file ‘SI_diffexp_all’, we report the assignment of each one of the 12,873 genes to a temporal pattern, by calculating the maximal similarity (Pearson correlation coefficient) to the average profile of each of the 9 clusters previously identified. Promoter binding analysis We collected all peak files available at the website of the ENCODE project [55] ( www.encodeproject.org ) for all members of the FOX proteins plus GATA1 as an outgroup. Peak files were calculated by the consortium using the peak caller MACS [56] on ChiPseq experiments done in duplicates, under standardized conditions. For the promoter binding analysis, (1) we took only peaks in common between the two duplicates by calculating the intersection of peaks with bedtools [57] ; (2) for each gene, we identified the promoter region as the genomic region 2000 bases upstream and 100 bases downstream of the transcription start site; (3) we counted peaks inside the promoter regions; (4) we calculated the proportion of genes having at least one peak in the promoter region, dividing the genes in downregulated (down), upregulated (up) and not differentially expressed (not de); (5) we divided the three proportions so obtained by the respective value of the not de group for each data set separately; and (6) the normalized proportion values of all data sets relative to the same transcription factor were averaged. For all the above steps, we considered as differentially expressed genes with FDR<0.01 and logFC>0.3 (or<0.3) at 3 h. P- values were determined using the non-parametric χ 2 -test for proportions (function prop.test) implemented in the R software ( http://www.r-project.org ). FOXM1 knockdown comparison The categories ‘up_drug’ and ‘down_drug’ refer to genes up- (logFC>0.5) and downregulated (logFC<−0.5) after 3 h treatment with FDI-6 , as measured by RNA-seq. The categories ‘up_kd’ and ‘down_kd’ refer to genes up- (logFC>0.5) and downregulated (logFC<−0.5) on FOXM1 knockdown, as measured by Affymetrix expression array ( http://www.ncbi.nlm.nih.gov/geo/query/acc.cgi?acc=GSE2222 ). ‘cluster5_down’ and ‘cluster5_up’ refers to genes downregulated (logFC<−0.5) belonging to cluster 5 from the temporal clustering analysis. P- values were determined using the non-parametric χ 2 -test for proportions (function prop.test) implemented in the R software ( http://www.r-project.org ). Motif analysis Fasta sequences from the genomic intervals corresponding to peaks were analysed by using the MEME-ChIP tool [58] from the MEME Suite for motif-based sequence analysis ( http://meme.nbcr.net/ ) and enriched motifs were identified ( Supplementary Fig. 9 ). General chemistry experimental methods Preparative purification was run on a Waters semi-preparative HPLC system using a Phenomenex Luna C18 (5 μm, 30 × 75 mm) at a flow rate of 45 ml min −1 . A gradient of 10% to 50% acetonitrile in water over 8 min (each containing 0.1% trifluoroacetic acid) was used as a mobile phase during the purification. Fraction collection was triggered by ultraviolet detection (220 nm). Analytical analysis was performed on an Agilent LC/MS (Agilent Technologies, Santa Clara, CA). Method 1: A 7 min gradient of 4% to 100% Acetonitrile (containing 0.025% trifluoroacetic acid) in water (containing 0.05% trifluoroacetic acid) was used with an 8 min run time at a flow rate of 1 ml min −1 . A Phenomenex Luna C18 column (3 μm, 3 × 75 mm) was used at a temperature of 50 °C. Method 2: A 3 min gradient of 4% to 100% Acetonitrile (containing 0.025% trifluoroacetic acid) in water (containing 0.05% trifluoroacetic acid) was used with a 4.5 min run time at a flow rate of 1 ml min −1 . A Phenomenex Gemini Phenyl column (3 μm, 3 × 100 mm) was used at a temperature of 50 °C. Purity was determined using an Agilent Diode Array Detector for both Method 1 and Method 2. Mass determination was performed using an Agilent 6130 mass spectrometer with electrospray ionization in the positive mode. 1 H NMR spectra were recorded on a Varian 400 MHz spectrometer. Chemical shifts are reported in ppm with undeuterated DMSO- d 6 at 2.49 p.p.m. as internal standard. High-resolution mass spectrometry was recorded on an Agilent 6210 Time-of-Flight LC/MS system. Confirmation of molecular formula was accomplished using electrospray ionization in the positive mode with the Agilent Masshunter software (version B.02). Synthesis of FDI-6 A mixture of 6-(thiophen-2-yl)-2-thioxo-4-(trifluoromethyl)-1,2-dihydropyridine-3-carbonitrile [59] (0.2 g, 0.699 mmol, 1 eq) and 2-chloro- N -(4-fluorophenyl)acetamide (0.138 g, 0.734 mmol, 1.05 eq) in ethanol (4 ml) was added to potassium carbonate (0.241 g, 1.746 mmol). The reaction mixture was refluxed for 4 h then poured into ice water. The precipitate was collected by filtration and washed with water. The crude solid was taken up in 3 ml DMSO and purified on a preparative HPLC to obtain pure FDI-6 as a TFA salt. LC-MS retention time: (Method 1)=7.081 min and (Method 2)=3.983 min; 1 H NMR (400 MHz, DMSO- d 6 ) δ 9.80 (s, 1H), 8.30 (s, 1H), 8.22 (dd, J =3.8, 1.1 Hz, 1H), 7.85 (dd, J =5.0, 1.1 Hz, 1H), 7.73–7.63 (m, 2H), 7.27 (dd, J =5.0, 3.8 Hz, 1H), 7.24–7.14 (m, 2H), 6.77 (s, 2H); 13C NMR (101 MHz, DMSO- d 6 ) δ 163.5, 160.5, 159.8, 157.4, 152.3, 145.1, 142.0, 134.7, 134.7, 131.7, 131.2, 129.1, 129.1, 123.7, 123.6, 117.8, 115.2, 114.9, 112.6, 100.7; HRMS (ESI) m/z (M+H)+ calcd. for C 19 H 12 F 4 N 3 OS 2 , 438.0352; found 438.367. Accession codes: RNA-seq profiling GEO: GSE58626. How to cite this article: Gormally, M. V. et al. Suppression of the FOXM1 transcriptional programme via novel small molecule inhibition. Nat. Commun. 5:5165 doi: 10.1038/ncomms6165 (2014).